SIRT6 represses LINE1 retrotransposons by ribosylating KAP1 but this repression fails with stress and age L1 retrotransposons are an abundant class of transposable elements that pose a threat to genome stability and may have a role in age-related pathologies such as cancer. Recent evidence indicates that L1s become more active in somatic tissues during the course of ageing; however the mechanisms underlying this phenomenon remain unknown. Here we report that the longevity regulating protein, SIRT6, is a powerful repressor of L1 activity. Specifically, SIRT6 binds to the 5′-UTR of L1 loci, where it mono-ADP ribosylates the nuclear corepressor protein, KAP1, and facilitates KAP1 interaction with the heterochromatin factor, HP1α, thereby contributing to the packaging of L1 elements into transcriptionally repressive heterochromatin. During the course of ageing, and also in response to DNA damage, however, we find that SIRT6 is depleted from L1 loci, allowing the activation of these previously silenced retroelements. Retrotransposons comprise a significant fraction of mammalian genomes [1] , [2] and are potent mediators of genomic instability [3] , [4] . Long interspersed element 1 (L1) retrotransposon activity, in particular, has been linked to DNA damage [5] , mutagenesis [6] , [7] and deregulation of host gene transcription [8] . Historically, retrotransposons were believed to be active only in germ cells, being subject to epigenetic silencing in somatic tissues. Recently, however, evidence has begun to accumulate indicating that the mechanisms that silence retrotransposons in somatic cells are not completely efficient [9] and may deteriorate with age [10] , [11] . Consistent with this observation, L1 activity has been implicated in a variety of age-related disorders [12] , including cancer [7] , [13] and neurodegeneration [14] , [15] . Given the emerging link between L1 activity and ageing, we hypothesized that the protein deacylase and mono-ADP ribosyltransferase enzyme, Sirtuin 6 (SIRT6), may function as an important L1 antagonist. Several mouse models have suggested that SIRT6 is a key regulator of mammalian lifespan. SIRT6 knockout (KO) mice develop a severe premature ageing syndrome, characterized by genomic instability, curvature of the spine, decreased bone mineral density, hypoglycemia and a severely shortened lifespan [16] . By contrast, mice overexpressing SIRT6 exhibit extended mean and median lifespans, concomitant with improved metabolic function [17] and cancer resistance [18] . At the molecular level, SIRT6 promotes longevity through multiple biological pathways. In particular, SIRT6 promotes DNA double-strand break repair [19] , [20] , regulates telomere stability [21] , suppresses inflammation [22] and opposes tumorigenesis [23] , [24] . In this study, we identify a new function for SIRT6 that may be relevant in the context of ageing. Here we report that SIRT6 is a powerful suppressor of L1 retrotransposon activity. Specifically, SIRT6 regulates the packaging of L1 elements into transcriptionally repressive heterochromatin by mono-ADP ribosylating the nuclear corepressor protein, KAP1 (KRAB-associated protein 1). Interestingly, however, we find that SIRT6 is depleted from L1 loci during the course of ageing and in response to genotoxic stressors, leading to the derepression of L1 elements. This suggests a paradigm by which L1s can become more active during the course of biological ageing and can contribute to the pathology of age-related diseases. SIRT6 is a powerful suppressor of L1 activity To examine whether SIRT6 has a role in suppressing L1 retrotransposition, we used a L1-enhanced green fluorescent protein (EGFP) reporter cassette [25] ( Supplementary Fig. 1 ) to measure de novo retrotransposition events in wild-type (WT) and SIRT6 KO cells. Deletion of SIRT6 resulted in a 3.3-fold increase in L1 retrotransposition frequency ( Fig. 1a ). Moreover, overexpression of SIRT6 in WT cells was sufficient to repress L1 retrotransposition frequency by 71% ( Fig. 1b ). Because SIRT6 is a chromatin-associated protein [26] , we hypothesized that SIRT6 may attenuate L1 activity by preventing transcription of L1 loci. Consistent with this hypothesis, L1 mRNA levels were elevated nearly fivefold in SIRT6 KO cells ( Fig. 1c ) and tissues ( Fig. 1d ); similarly, depletion of SIRT6 in human dermal fibroblasts (HDF cells) with SIRT6-targeting short hairpin RNAs resulted in a 4.4-fold increase in L1 expression ( Supplementary Fig. 2 ). We also observed an increase in the transcriptional activity of several other repetitive elements, including Alu elements and minor satellite repeats ( Supplementary Fig. 3 ). Because of the particularly deleterious effects that L1 elements can have on genome stability, we focused our attention on understanding how SIRT6 suppresses the activity of this family of elements. Finally, using a sensitive quantitative PCR (qPCR) method for detecting de novo retroelement insertions [27] , we found that SIRT6 KO mouse embryonic fibroblasts (MEFs) had elevated genomic L1 DNA content, indicating that retrotransposition events occur more frequently in SIRT6 KO cells, relative to WT ( Fig. 1e ). 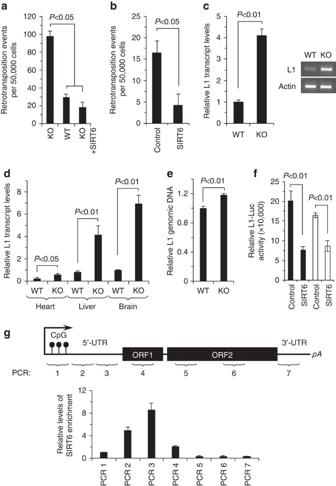Figure 1: SIRT6 mediates the transcriptional silencing of L1 loci. (a) L1 retrotransposition activity is elevated in SIRT6 KO cells. WT and SIRT6 KO MEFs were transfected with a L1-EGFP reporter plasmid (Supplementary Fig. 1). GFP-positive cells, indicatingde novoretrotransposition events, were scored by fluorescence-activated cell sorting. This experiment was repeated five times, error bars indicate s.d. (b) Overexpression of SIRT6 is sufficient to suppress L1 retrotransposition in HDF cells, as measured using the L1-EGFP reporter assay. Cells were transfected with 5 μg of the L1-EGFP reporter and either a control (HPRT) or SIRT6-encoding plasmid;n=3, error bars indicate s.d. (c) L1 mRNA is more abundant in SIRT6 KO cells than WT cells. Total cellular RNA was extracted from WT and SIRT6 KO MEFs. L1 mRNA was quantified by qRT–PCR; quantification was normalized to actin mRNA levels;n=4, error bars indicate s.d. (d) L1 mRNA is more abundant in the tissues of SIRT6 KO mice than the tissues of WT littermates. Total cellular RNA was extracted from the indicated tissues of WT and SIRT6 KO mice. L1 mRNA was quantified by qRT–PCR, L1 expression was normalized to actin expression;n=4, error bars indicate s.d. (e) MEFs in the SIRT6 KO background had higher L1 ORF2 DNA content than WT cells. L1 copy number was probed using qPCR with primers spanning ORF2, and normalized to 5S genomic content;n=3, error bars indicate s.d. (f) SIRT6 represses transcription of the L1 5′-UTR. A L1-5′-UTR reporter was either transiently transfected (black bars) or chromosomally integrated (open bars) into HDF cells. Overexpression of SIRT6 in these cells repressed the transcriptional activity of the L1 5′-UTR by ~55–70%, relative to control, HPRT overexpression, experiments.N=5, error bars indicate s.d. (g) SIRT6 localizes to the 5′-UTR of endogenous L1 elements in the genome. ChIP was performed using the indicated antibodies and primers spanning the indicated regions of the L1 locus. Representative ChIP experiment results are shown, the ChIP was repeated three times. Where appropriate, statistical significance was determined by use of the Student’st-test. Figure 1: SIRT6 mediates the transcriptional silencing of L1 loci. ( a ) L1 retrotransposition activity is elevated in SIRT6 KO cells. WT and SIRT6 KO MEFs were transfected with a L1-EGFP reporter plasmid ( Supplementary Fig. 1 ). GFP-positive cells, indicating de novo retrotransposition events, were scored by fluorescence-activated cell sorting. This experiment was repeated five times, error bars indicate s.d. ( b ) Overexpression of SIRT6 is sufficient to suppress L1 retrotransposition in HDF cells, as measured using the L1-EGFP reporter assay. Cells were transfected with 5 μg of the L1-EGFP reporter and either a control (HPRT) or SIRT6-encoding plasmid; n =3, error bars indicate s.d. ( c ) L1 mRNA is more abundant in SIRT6 KO cells than WT cells. Total cellular RNA was extracted from WT and SIRT6 KO MEFs. L1 mRNA was quantified by qRT–PCR; quantification was normalized to actin mRNA levels; n =4, error bars indicate s.d. ( d ) L1 mRNA is more abundant in the tissues of SIRT6 KO mice than the tissues of WT littermates. Total cellular RNA was extracted from the indicated tissues of WT and SIRT6 KO mice. L1 mRNA was quantified by qRT–PCR, L1 expression was normalized to actin expression; n =4, error bars indicate s.d. ( e ) MEFs in the SIRT6 KO background had higher L1 ORF2 DNA content than WT cells. L1 copy number was probed using qPCR with primers spanning ORF2, and normalized to 5S genomic content; n =3, error bars indicate s.d. ( f ) SIRT6 represses transcription of the L1 5′-UTR. A L1-5′-UTR reporter was either transiently transfected (black bars) or chromosomally integrated (open bars) into HDF cells. Overexpression of SIRT6 in these cells repressed the transcriptional activity of the L1 5′-UTR by ~55–70%, relative to control, HPRT overexpression, experiments. N =5, error bars indicate s.d. ( g ) SIRT6 localizes to the 5′-UTR of endogenous L1 elements in the genome. ChIP was performed using the indicated antibodies and primers spanning the indicated regions of the L1 locus. Representative ChIP experiment results are shown, the ChIP was repeated three times. Where appropriate, statistical significance was determined by use of the Student’s t -test. Full size image SIRT6 regulates packaging of L1s into heterochromatin L1 transcription is driven by an internal promoter within the L1 5′-untranslated region (UTR). To test whether SIRT6 directly regulates L1 transcription, we cloned the human L1 5′-UTR into a luciferase reporter plasmid. Overexpression of SIRT6 strongly repressed signalling from this reporter, both in an episomal and chromosomally integrated context ( Fig. 1f ). The efficiency with which SIRT6 mediated the silencing of the L1 5′-UTR was similar to the efficiency with which SIRT6 repressed other known SIRT6-regulated genes ( Supplementary Fig. 4 ). To gain insight into how SIRT6 may be regulating the transcriptional silencing of L1s, we analysed data sets from SIRT6 chromatin immunoprecipitation (ChIP) followed by massively parallel DNA sequencing experiments [28] . We observed that L1 5′-UTR sequences were heavily represented in the SIRT6 ChIP-sequencing (ChIP-seq) data set ( Supplementary Fig. 5 ). We confirmed that SIRT6 localized to L1 loci in HDF cells by ChIP, and observed that SIRT6 was specifically enriched at the 5′-UTR of L1 loci ( Fig. 1g ). Cumulatively, these results led us to speculate that SIRT6 attenuates L1 transcription by modulating the heterochromatin status of the L1 promoter. Micrococcal nuclease digestion of genomic DNA from WT and SIRT6 KO MEFs revealed that in the absence of SIRT6, higher-order chromatin structures are significantly perturbed ( Fig. 2a ). While this appeared to be a global feature of the SIRT6 KO genome, closer examination revealed that L1 loci were particularly sensitive to micrococcal nuclease treatment ( Supplementary Fig. 6 ). Consistent with this observation, L1 loci exhibited multiple signs of failure to form constitutive heterochromatin in SIRT6 KO cells. In particular, the CpG island within the L1 5′-UTR was hypomethylated ( Fig. 2b ) and the constitutive heterochromatin marker, histone H3 trimethylated at Lys9, was significantly depleted from the endogenous L1 5′-UTR in SIRT6 KO cells ( Fig. 2c and Supplementary Fig. 7a ). Moreover, the heterochromatin regulating proteins MeCP2 (methyl CpG binding protein 2) and KAP1 were also depleted from the L1 5′-UTR in SIRT6 KO cells ( Fig. 2c and Supplementary Fig. 7b,c ). Consistent with a role for SIRT6 in regulating heterochromatin formation, we observed that SIRT6 interacts with multiple heterochromatin proteins, including KAP1, HP-1α (heterochromatin protein 1 alpha) and MeCP2 ( Fig. 2d ), and that these interactions were independent of DNA ( Supplementary Fig. 8 ). Cumulatively, these results indicate that SIRT6 is required for packaging L1 loci into transcriptionally repressive heterochromatin. 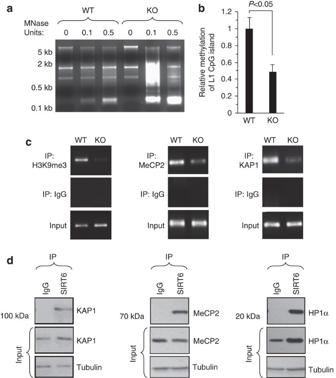Figure 2: In the absence of SIRT6 heterochromatin is perturbed at L1 sites. (a) Higher-order heterochromatin is disrupted in the genome of SIRT6 KO mice. Whole-genomic DNA was extracted from WT and SIRT6 KO cells, and then digested with the indicated units of micrococcal nuclease (MNase). Digested DNA was separated by gel electrophoresis. This experiment was repeated three times and a representative result is shown. (b) The L1 5′-UTR is hypomethylated in SIRT6 KO cells. Whole-genomic DNA was extracted from SIRT6 KO and WT fibroblasts; methylation levels were quantified using bisulphite primers following bisulphite conversion;n=3, error bars indicate s.d. (c) Multiple heterochromatin formation and maintenance proteins, namely H3K9me3, MeCP2 and KAP1 are specifically depleted from the L1 5′-UTR in SIRT6 KO cells. ChIP was performed using the indicated antibodies in WT and SIRT6 KO cells. Primers spanning the mouse L1 5′-UTR were used for quantification. These experiments were performed three times and representative results are shown. Quantification of the data by qPCR is shown inSupplementary Fig. 5. (d) SIRT6 interacts with multiple heterochromatin associated proteins, including KAP1, MeCP2 and HP1α. SIRT6 was immunoprecipitated from HDF cells and the precipitate was probed with the indicated antibodies. These experiments were repeated three times and representative blots are shown; Input was loaded at 5%. Where appropriate, statistical significance was determined by use of the Student’st-test. Figure 2: In the absence of SIRT6 heterochromatin is perturbed at L1 sites. ( a ) Higher-order heterochromatin is disrupted in the genome of SIRT6 KO mice. Whole-genomic DNA was extracted from WT and SIRT6 KO cells, and then digested with the indicated units of micrococcal nuclease (MNase). Digested DNA was separated by gel electrophoresis. This experiment was repeated three times and a representative result is shown. ( b ) The L1 5′-UTR is hypomethylated in SIRT6 KO cells. Whole-genomic DNA was extracted from SIRT6 KO and WT fibroblasts; methylation levels were quantified using bisulphite primers following bisulphite conversion; n =3, error bars indicate s.d. ( c ) Multiple heterochromatin formation and maintenance proteins, namely H3K9me3, MeCP2 and KAP1 are specifically depleted from the L1 5′-UTR in SIRT6 KO cells. ChIP was performed using the indicated antibodies in WT and SIRT6 KO cells. Primers spanning the mouse L1 5′-UTR were used for quantification. These experiments were performed three times and representative results are shown. Quantification of the data by qPCR is shown in Supplementary Fig. 5 . ( d ) SIRT6 interacts with multiple heterochromatin associated proteins, including KAP1, MeCP2 and HP1α. SIRT6 was immunoprecipitated from HDF cells and the precipitate was probed with the indicated antibodies. These experiments were repeated three times and representative blots are shown; Input was loaded at 5%. Where appropriate, statistical significance was determined by use of the Student’s t -test. Full size image SIRT6 mono-ADP ribosylates KAP1 to promote L1 silencing SIRT6 has multiple biochemical activities, including protein deacetylation [22] and mono-ADP ribosylation [19] , [29] . To determine which of these activities was required to mediate L1 silencing, we transfected cells with SIRT6 expression vectors in which key catalytic residues had been mutated [19] such that the enzyme could catalyse only deacetylation reactions (SIRT6 G60A), only mono-ADP ribosylation reactions (SIRT6 R65A) or neither (SIRT6 S56Y). Only the mono-ADP ribosylation activity of SIRT6 was required to abrogate the transcriptional activity of L1 elements ( Fig. 3a ). Consistent with this observation, we observed that acetylation of SIRT6 deacetylation targets, H3K9ac and H3K56ac, was only slightly elevated at L1 loci in SIRT6 KO cells ( Supplementary Fig. 9a,b ). SIRT6 has been reported to mono-ADP ribosylate PARP1 (ref. 19 ), a protein which has been implicated in the silencing of retrotransposons in Drosophila [30] ; however, in our system, PARP1 was dispensable for SIRT6-mediated silencing of L1s ( Supplementary Fig. 10 ). Because we had observed that SIRT6 interacts with KAP1, HP1α and MeCP2 via co-immunoprecipitation (co-IP), we tested whether SIRT6 could mono-ADP ribosylate any of these proteins in vitro . SIRT6 transferred radiolabelled NAD + to KAP1, but not to any other substrate tested ( Fig. 3b ). Depletion of KAP1 from HDF cells by short hairpin RNA resulted in a threefold increase in L1 transcriptional activity, phenocopying SIRT6 depletion ( Fig. 3c ); overexpression of KAP1 was also sufficient to reduce L1 transcription by 20% ( Supplementary Fig. 11 ). Importantly, overexpression of SIRT6 in KAP1-depleted HDF cells failed to induce L1 silencing, indicating that KAP1 is required for SIRT6 to induce heterochromatinization of L1 loci ( Fig. 3d ). KAP1 has been reported to induce silencing of endogenous retroelements [31] in part by coordinating the assembly of a HP1α-SETDB1-dependent corepressor complex [32] . Using co-IP to probe for interactions between KAP1 and these proteins, we found that SIRT6 did not modulate interactions between KAP1 and SETDB1 ( Supplementary Fig. 12 ). Instead, we noted that in the absence of SIRT6, the interaction between KAP1 and HP1α was strongly abrogated ( Fig. 3e ). Overexpression of WT SIRT6 and SIRT6 R65A was sufficient to restore KAP1–HP1α interactions to WT levels; in contrast, overexpression of SIRT6 G60A or SIRT6 S56Y failed to restore KAP1–HP1α interactions ( Fig. 3e ). Similarly, overexpression of SIRT6 and SIRT6 R65A was sufficient to restore enrichment of KAP1, HP1α and H3K9me3 at L1 loci to WT levels in SIRT6 KO cells ( Supplementary Fig. 13a–c ). Finally, using an in vitro IP system, we observed that WT SIRT6 and SIRT6 R65A, but not SIRT6 G60A or SIRT6 S56Y, strongly stimulated binding between KAP1 and HP1α ( Fig. 3f ). Cumulatively, these results suggest that ribosylation of KAP1 by SIRT6 is required for efficient silencing of L1 retrotransposons. KAP1 is known to suppress the expression of other retroelements, in particular intracisternal A-type particles (IAP), and to regulate gene expression at a wide range of loci. We observed that SIRT6 also appears to regulate IAP expression, with IAP transcript levels elevated in SIRT6 KO cells. However, analysis of promoter arrays [41] , [42] showed that SIRT6 only co-occupies ~10% of KAP1 bound promoters, suggesting that SIRT6 and Kap1 cooperate to suppress retroelements but have divergent functions in regulation of gene expression ( Supplementary Fig. 14a–c ). 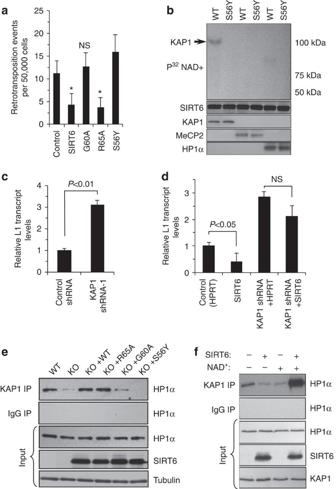Figure 3: SIRT6 mono-ADP ribosylates KAP1 to induce L1 silencing. (a) The mono-ADP ribosylation activity of SIRT6 is required to mediate L1 transcriptional silencing. HDF cells were transfected with the L1-EGFP reporter plasmid and the indicated expression vector. Retrotransposition events were scored by fluorescence-activated cell sorting, asterisk indicatesP>0.05 when compared with control,n=5; NS, not significant. (b) SIRT6 mono-ADP ribosylates KAP1, but not MeCP2 or HP1α. WT or catalytically inactive (S56Y) SIRT6 was incubated with the indicated substrates in the presence of radiolabelled NAD+. Mono-ADP ribosylation was detected by transfer of the radiolabel to the substrate. This experiment was repeated three times and a representative result is shown. (c) Depletion of KAP1 by short hairpin RNA in HDF cells phenocopies SIRT6 depletion. Cells were stably transfected with either control or KAP1 targeting short hairpin RNAs (Supplementary Fig. 6B); L1 mRNA levels were quantified by qRT-PCR;n=3, error bars indicate s.d. (d) SIRT6 fails to silence L1 transcription in the absence of KAP1. SIRT6 overexpression was not sufficient to reduce L1 transcription in KAP1-depleted cells;n=3, error bars indicate s.d.; NS, not significant. (e) In the absence of SIRT6, KAP1 does not stably interact with HP1α. KAP1 was immunoprecipitated from WT, SIRT6 KO and SIRT6 KO expressing WT SIRT6 or SIRT6 activity mutants (R65A, ribosylation only; G60A, deacetylation only; S56Y, catalytically dead) cells and then probed with HP1α antibodies. This experiment was repeated three times and a representative result is shown. (f) SIRT6 promotes interaction between KAP1 and HP1α. KAP1 was incubated in the presence or absence of SIRT6 or SIRT6 activity mutants before addition of HP1α and PCR-amplified L1 5′-UTR. KAP1 was immunoprecipitated from each reaction and its affinity for HP1α was quantified by immunoblot. This experiment was repeated three times and a representative result is shown. Where appropriate, statistical significance was determined by use of the Student’st-test. Figure 3: SIRT6 mono-ADP ribosylates KAP1 to induce L1 silencing. ( a ) The mono-ADP ribosylation activity of SIRT6 is required to mediate L1 transcriptional silencing. HDF cells were transfected with the L1-EGFP reporter plasmid and the indicated expression vector. Retrotransposition events were scored by fluorescence-activated cell sorting, asterisk indicates P >0.05 when compared with control, n =5; NS, not significant. ( b ) SIRT6 mono-ADP ribosylates KAP1, but not MeCP2 or HP1α. WT or catalytically inactive (S56Y) SIRT6 was incubated with the indicated substrates in the presence of radiolabelled NAD + . Mono-ADP ribosylation was detected by transfer of the radiolabel to the substrate. This experiment was repeated three times and a representative result is shown. ( c ) Depletion of KAP1 by short hairpin RNA in HDF cells phenocopies SIRT6 depletion. Cells were stably transfected with either control or KAP1 targeting short hairpin RNAs ( Supplementary Fig. 6B ); L1 mRNA levels were quantified by qRT-PCR; n =3, error bars indicate s.d. ( d ) SIRT6 fails to silence L1 transcription in the absence of KAP1. SIRT6 overexpression was not sufficient to reduce L1 transcription in KAP1-depleted cells; n =3, error bars indicate s.d. ; NS, not significant. ( e ) In the absence of SIRT6, KAP1 does not stably interact with HP1α. KAP1 was immunoprecipitated from WT, SIRT6 KO and SIRT6 KO expressing WT SIRT6 or SIRT6 activity mutants (R65A, ribosylation only; G60A, deacetylation only; S56Y, catalytically dead) cells and then probed with HP1α antibodies. This experiment was repeated three times and a representative result is shown. ( f ) SIRT6 promotes interaction between KAP1 and HP1α. KAP1 was incubated in the presence or absence of SIRT6 or SIRT6 activity mutants before addition of HP1α and PCR-amplified L1 5′-UTR. KAP1 was immunoprecipitated from each reaction and its affinity for HP1α was quantified by immunoblot. This experiment was repeated three times and a representative result is shown. Where appropriate, statistical significance was determined by use of the Student’s t -test. Full size image SIRT6 vacates L1 loci during ageing and in response to stress Several reports have implicated retrotransposons as drivers of phenotypes associated with the ageing process [11] , [33] , [34] . To examine whether L1 retrotransposons, the most active members of the mammalian retrotransposon family, are relevant in this context, we used quantitative reverse transcription PCR (qRT–PCR) to quantify L1 mRNA levels in young and replicatively senescent human fibroblasts ( Supplementary Fig. 15 ). Senescent cells, which have been implicated in the aetiology of ageing [35] , exhibited a 3.1-fold increase in L1 mRNA levels ( Fig. 4a ). We also examined L1 expression in brain, liver and heart tissue from young (4 months old) and old (24 months old) mice. Of the organs analysed, the brain exhibited the most significant deregulation of L1 expression with age (7.1-fold increased L1 expression in old brain tissue, relative to young brain tissue), liver tissue exhibited a modest increase in L1 expression with age (65% increase) and heart tissue exhibited a non-significant decline in L1 expression with age ( Fig. 4b ). ChIP analysis revealed that SIRT6 was depleted from the L1 5′-UTR in senescent cells ( Fig. 4c ) and also in old brain tissue ( Fig. 4d and Supplementary Fig. 16a,b ), suggesting that vacation of the L1 5′-UTR by SIRT6 may be driving this phenotype. We also observed that SIRT6 was only slightly depleted from the L1 5′-UTR in liver tissue and not significantly depleted from the L1 5′-UTR in heart tissue ( Supplementary Fig. 17 )—two tissues that did not exhibit large age-dependent changes in L1 expression ( Fig. 4b ). Consistent with this hypothesis, overexpression of SIRT6 in senescent cells was sufficient to partially restore L1 expression to youthful levels ( Fig. 4e ). 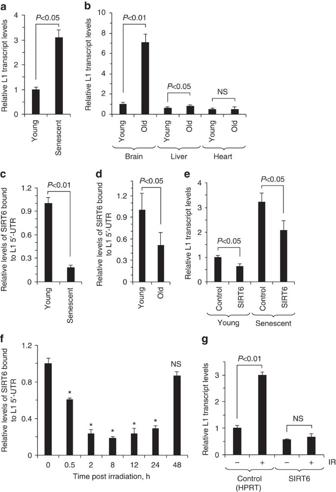Figure 4: SIRT6 vacates L1 promoters in aged cells leading to derepression of L1. (a) Senescent cells exhibit elevated L1 expression. Total cellular RNA was isolated from young and replicatively senescent HDF cells. L1 levels were quantified by qRT–PCR and normalized to actin expression;n=5, error bars indicate s.d. (b) Brain and liver tissue from old mice exhibits increased L1 expression. Total RNA was isolated from the indicated tissues from young (4 months old) and old (24 months old) mice. L1 levels were quantified by qRT–PCR and normalized to actin expression;n=3, error bars indicate s.d.; NS, not significant. (c) SIRT6 is depleted from the L1 5′-UTR in senescent cells. ChIP with SIRT6 antibodies revealed that the protein is depleted from the L1 5′-UTR in senescent cells, relative to young cells. Relative enrichment, after normalization to input and H3 levels is shown;n=3, error bars indicate s.d. (d) SIRT6 is depleted from the L1 5′-UTR in old brain tissue. ChIP with SIRT6 antibodies revealed that the protein is depleted from the L1 5′-UTR in old brain tissue, relative to young brain tissue. Relative enrichment, after normalization to input and H3 levels is shown;n=3, error bars indicate s.d. (e) Overexpression of SIRT6 partially restores L1 expression to youthful levels in senescent cells. Young and senescent cells were transfected with either a HRPT- or SIRT6-encoding expression plasmid. Total RNA was isolated from these cells and L1 expression was quantified by qRT–PCR after normalization to actin expression;n=3, error bars indicate s.d. (f) DNA damage is sufficient to rapidly induce SIRT6 relocalization. ChIP-qPCR with SIRT6 antibodies revealed that the protein is rapidly depleted from the L1 5′-UTR in response to gamma irradiation. (g) Overexpression of SIRT6 attenuates gamma irradiation induced activation of L1 transcription. Cells were transfected with the indicated vector and then irradiated with gamma irradiation. L1 levels were quantified by qRT–PCR;n=3, error bars indicate s.d.; NS, not significant. Where appropriate, statistical significance was determined by the Student’st-test. Figure 4: SIRT6 vacates L1 promoters in aged cells leading to derepression of L1. ( a ) Senescent cells exhibit elevated L1 expression. Total cellular RNA was isolated from young and replicatively senescent HDF cells. L1 levels were quantified by qRT–PCR and normalized to actin expression; n =5, error bars indicate s.d. ( b ) Brain and liver tissue from old mice exhibits increased L1 expression. Total RNA was isolated from the indicated tissues from young (4 months old) and old (24 months old) mice. L1 levels were quantified by qRT–PCR and normalized to actin expression; n =3, error bars indicate s.d. ; NS, not significant. ( c ) SIRT6 is depleted from the L1 5′-UTR in senescent cells. ChIP with SIRT6 antibodies revealed that the protein is depleted from the L1 5′-UTR in senescent cells, relative to young cells. Relative enrichment, after normalization to input and H3 levels is shown; n =3, error bars indicate s.d. ( d ) SIRT6 is depleted from the L1 5′-UTR in old brain tissue. ChIP with SIRT6 antibodies revealed that the protein is depleted from the L1 5′-UTR in old brain tissue, relative to young brain tissue. Relative enrichment, after normalization to input and H3 levels is shown; n =3, error bars indicate s.d. ( e ) Overexpression of SIRT6 partially restores L1 expression to youthful levels in senescent cells. Young and senescent cells were transfected with either a HRPT- or SIRT6-encoding expression plasmid. Total RNA was isolated from these cells and L1 expression was quantified by qRT–PCR after normalization to actin expression; n =3, error bars indicate s.d. ( f ) DNA damage is sufficient to rapidly induce SIRT6 relocalization. ChIP-qPCR with SIRT6 antibodies revealed that the protein is rapidly depleted from the L1 5′-UTR in response to gamma irradiation. ( g ) Overexpression of SIRT6 attenuates gamma irradiation induced activation of L1 transcription. Cells were transfected with the indicated vector and then irradiated with gamma irradiation. L1 levels were quantified by qRT–PCR; n =3, error bars indicate s.d. ; NS, not significant. Where appropriate, statistical significance was determined by the Student’s t -test. Full size image SIRT6 is known to rapidly relocalize to DNA damage sites in response to oxidative stress [19] , [36] . We hypothesized that such stress may deplete SIRT6 from the L1 5′-UTR, creating a window for increased L1 activity. Treating cells with either gamma irradiation or hydrogen peroxide induced rapid mobilization of SIRT6 away from the L1 5′-UTR and resulted in increased L1 expression ( Fig. 4f and Supplementary Fig. 18 ). Overexpression of SIRT6 before exposure to genotoxic compounds was sufficient to prevent stress-induced activation of L1 elements ( Fig. 4g ). DNA damage is more abundant in old cells and tissues [37] , [38] . This suggests a paradigm wherein SIRT6 is normally localized to L1 loci, repressing their transcription by mono-ADP-ribosylating Kap1 and facilitating its interaction with HP1α; in response to stress, however, SIRT6 vacates these sites in order to facilitate DNA repair, creating a window for increased L1 activity, which could in part explain the age-related increase in L1 expression ( Fig. 5 ). 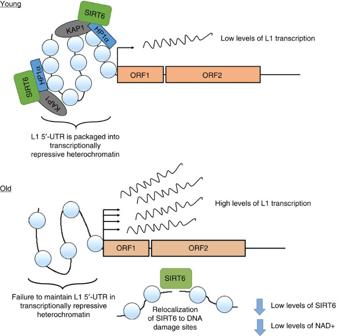Figure 5: Model for age-related derepression of L1. In young cells, L1s are maintained in a silent state. SIRT6 has a critical role in regulating the transcriptional repression of L1s in young cells by coordinating the packaging of the L1 5′-UTR into transcriptionally repressive heterochromatin. In old and senescent cells, however, L1s become more active. This derepression of L1s in is part owing to a failure in maintaining the L1 5′-UTR in a constitutively heterochromatic state. This failure to properly package the L1 5′-UTR in heterochromatin stems from depletion of SIRT6 from the L1 5′-UTR. Old and senescent cells accumulate DNA damage, causing SIRT6 to relocalize from the L1 5′-UTR to DNA damage sites where it coordinates DNA repair. As a result of this relocalization, however, the repressive machinery at the L1 5′-UTR becomes less efficient, allowing for activation of L1 elements. Additional factors that may contribute to reduced SIRT6-mediated L1 silencing are declining levels of nuclear NAD+56and lower levels of SIRT6 in senescent cells57. Figure 5: Model for age-related derepression of L1. In young cells, L1s are maintained in a silent state. SIRT6 has a critical role in regulating the transcriptional repression of L1s in young cells by coordinating the packaging of the L1 5′-UTR into transcriptionally repressive heterochromatin. In old and senescent cells, however, L1s become more active. This derepression of L1s in is part owing to a failure in maintaining the L1 5′-UTR in a constitutively heterochromatic state. This failure to properly package the L1 5′-UTR in heterochromatin stems from depletion of SIRT6 from the L1 5′-UTR. Old and senescent cells accumulate DNA damage, causing SIRT6 to relocalize from the L1 5′-UTR to DNA damage sites where it coordinates DNA repair. As a result of this relocalization, however, the repressive machinery at the L1 5′-UTR becomes less efficient, allowing for activation of L1 elements. Additional factors that may contribute to reduced SIRT6-mediated L1 silencing are declining levels of nuclear NAD + [56] and lower levels of SIRT6 in senescent cells [57] . Full size image In summary, we have demonstrated that the longevity protein, SIRT6, is a critical suppressor of L1 activity. Mechanistically, SIRT6 enforces the silencing of L1s by coordinating the packaging of these transposable elements into transcriptionally repressive heterochromatin. A main feature of this silencing process is the mono-ADP ribosylation of the nuclear corepressor protein, KAP1, by SIRT6. KAP1 is a pleiotropic regulator of a diverse range of cellular processes including gene silencing, cell growth and differentiation, pluripotency, apoptosis, DNA repair and maintenance of genomic integrity [39] . Of particular interest to this study, KAP1 is known to have a critical role in suppressing endogenous retroviruses and has recently emerged as a regulator of L1s as well [31] , [40] . KAP1 appears to enforce silencing by facilitating the recruitment of additional silencing factors at the target locus. Consistent with this model, we find that mono-ADP ribosylation of KAP1 by SIR6 is required for the recruitment of HP1α to L1 loci. Finally, it is worth noting that post-translational modification of KAP1 has a critical role in determining which cellular context the protein will function in, for example, sumoylated KAP1 promotes regulation of gene expression, whereas phosphorylated KAP1 promotes DNA repair [41] , [42] . Our data suggests that mono-ADP ribosylation of KAP1 may be critical for the suppression of transposable elements. In response to genotoxic stress, and during the course of ageing, we observed that SIRT6 is depleted from L1 loci, resulting in the upregulation of L1 activity. This relocalization of SIRT6 in response to stress is reminiscent of the ‘redistribution of chromatin modifier theory of ageing’ [43] , [44] , which predicts that while mobilization of chromatin modifying elements in response to stress–stimuli is adaptive in young organisms, constitutive redistribution of these elements may drive age-related phenotypes. In this context, derepression of L1 in response to SIRT6 mobilization to DNA damage sites represents a threat to genome stability and may be important in the manifestation of ageing. For example, by definition, the de novo insertions that result from L1 retrotransposition are mutagenic; in addition, the L1 ORF2 encodes an endonuclease that, when expressed, induces DNA damage; finally, massive L1 transcriptional activity itself can induce misregulation of gene expression and ‘clog’ the transcriptional machinery of the host—for these reasons, it is easy to envision how constitutive L1 activity can drive age-related pathologies. Indeed, overexpression of exogenous full-length L1 has been shown to induce a senescence-like phenotype in human fibroblasts and adult stem cells [9] . This reasoning is especially intriguing in conjunction with our observation that L1 activity in the brain is particularly sensitive to upregulation during ageing and in the absence of SIRT6. Several other reports have indicated that retrotransposition occurs more frequently in the brain, and, in particular, in the hippocampus and striatum, relative to other somatic tissues, such as blood, heart and liver [45] , [46] . Moreover, de novo insertions of retrotransposons appear to preferentially affect actively transcribed genes in the brain, including dopamine receptors, amino acid transporters and genes regulating synaptic transmission [45] . These observations have led to the hypothesis that deregulation of L1s may contribute to disease pathogenesis in the brain; consistent with this notion, several neurological disorders, including Rett syndrome, Smith–Magenis syndrome and schizophrenia are characterized by dysregulation of L1 activity [27] , [45] , [47] . Given our observations that L1 activity increases in aged brains, it is therefore tempting to speculate that deregulation of L1 silencing with age may also contribute to age-related pathologies of the nervous system, ranging from cancer to neurodegenerative disorders. Further studies will be required, however, to fully investigate this possibility. It is also worth noting that Sirtuin 1, another mammalian member of the siruin gene family, has been implicated in silencing repetitive elements, including retrotransposons and major satellite repeats [43] , [48] . It will be interesting to test whether Sirtuin 1 and SIRT6 operate through similar or divergent pathways to enforce the repression of repetitive elements. Cumulatively, this study builds on the mounting body of evidence that suggests that L1s become more transcriptionally active during ageing and senescence [10] , [49] , and provides a molecular mechanism to explain this phenomenon. While future studies will be required to delineate to what extent L1 hyperactivity drives age-related pathologies, our results lay the foundation for such research and encourages researchers to revise the old paradigm that L1 activity is primarily important in the context of the germ line. Mice and MEF cell lines SIRT6 KO and WT mice were obtained from Jackson Laboratories (strain number:129-Sirt6tm1Fwa/J, stock number: 006050). MEF cells were extracted from embryos using standard assay and genotyped using PCR and western blot. Specifically, day 14 embryos were dissected and heads were used for genotyping; the remainder of the tissue was minced with forceps and transferred to conical tubes containing 2 × trypsin. The tubes were incubated at 37 °C for 5 min. The digested tissue was then rinsed in prewarmed MEF media (DMEM, 10% fetal bovine serum and 1% penicillin/streptomycin) five times. Cells were then plated onto tissue culture plates and passaged when 70% confluent. Young (4 months old) and old (24 months old) female C57BL/6 WT mice, used for quantifying L1 expression in young and old tissues, were derived from our ageing colony. All animals were housed in accordance with regulations designated by the University of Rochester’s Committee on Use and Care of Animals approved protocols. Cell culture All cell lines used in this study were grown in a humidified incubator programmed to 5% CO 2 , 5% O 2 and 37 °C. HDF and MEF cells were grown in Eagle’s minimum essential medium with Earle’s salts supplemented with 15% fetal calf serum, nonessential amino acids, 1 mM sodium pyruvate and penicillin–streptomycin. Transfections Cells were split 2 days before transfection at a density of 500,000 cells per 10 cm plate. Transfection was then performed using the Amaxa Nucleofector machine (Lonza) and the Normal Human Dermal Fibroblast (NHDF) transfection solution. Plasmids and antibodies The episomal L1-EGFP reporter plasmid and the L1 5′-UTR luciferase reporter plasmid used in this study were both described previously [25] , [50] . Both constructs were kindly provided by John V. Moran. Plasmids encoding SIRT6, SIRT6 mutants, KAP1 and HPRT were cloned by amplifying the corresponding cDNA from HDF cells and then ligating the amplicon into a NotI/SalI digested pEGFP-N1 backbone. The following antibodies were used in this study: 1:500 SIRT6 (ab48352 and ab62739, Abcam), 1:500 KAP1 (ab10483, Abcam), 1:500 SETDB1 (ab12317, Abcam), 1:500 MeCP2 (ab2828, Abcam), 1:1,000 H3K9me3 (ab8898, Abcam) and 1:1,000 HP1α (mab3448, Millipore). Luciferase assay The luciferase assay using the L1-5′-UTR reporter has been previously described [50] . Briefly, HDF cells were transfected with the 3-μg L1-5′-UTR luciferase reporter and 5 μg of either an HPRT-encoding or SIRT6-encoding expression vector. Cells were allowed to recover for 48–72 h and then harvested for analysis. Experiments were repeated three times, in triplicate each time. Luciferase activity was normalized to the number of cells harvested. Cells expressing a stably integrated L1 5′-UTR luciferase reporter were constructed by linearizing 10 μg of L1-5′-UTR luciferase reporter by digestion with SalI, and transfecting immortalized human fibroblasts with the linearized DNA. The cells were passaged for 4 weeks to ensure that luciferase signal was generated by stably integrated L1-5′-UTR reporter. Chromatin immunoprecipitation ChIP assays were performed as per the manufacturer’s protocol (Abcam, ab500). Specifically, a minimum of 2 million cells were used for each reaction. SIRT6, H3K9me3, KAP1, MeCP2 and H3 antibodies were used to precipitate the proteins of interest; an IgG control was used for each precipitation experiment. After precipitation, chromatin fragments were amplified with primers spanning the L1 locus in order to quantify the relative binding of each of these proteins. Primer sequences: L1 PCR1 5′-AAGATGGCCGAATAGGAACAG-3′ (forward) and 5′-TTTGACTCGGAAAGGGAACTC-3′ (reverse), L1 PCR2 5′-ACGAGACTATATCCCACACCT-3′ (forward) and 5′-GCAGAGGTTACTGCTGTCTT (reverse), L1 PCR3 5′-TGTCTGACAGCTTTGAAGAGAG-3′ (forward) and 5′-TGGTCTTTGATGATGGTGATGTA-3′ (reverse), L1 PCR4 5′-CGATGCGATCAACTGGAAG-3′ (forward) and 5′-GGCCTGCCTTGCTAGATT-3′ (reverse), L1 PCR5 5′-CAGAGACACACATAGGCTCAAA-3′ (forward) and 5′-AATCTGGGTGCTCCTGTATTG-3′ (reverse), L1 PCR6 5′-ACTCATCTGACAAAGGGCTAAT-3′ (forward) and 5′-CCTATTTCTCCGCATCCTCTC-3′ (reverse), L1 PCR7 5′-AATGAGATCACATGGACACAGGAAG-3′ (forward) and 5′-TGTATACATGTGCCATGCTGGTGC-3′ (reverse). Mouse L1 5′-UTR forward: 5′-AGCTTCTGGAACAGGCAGAA-3′ and reverse: 5′-CACTGTGTTGCTTTGGCAGT-3′. Input was 5% for all samples. Relative protein binding was calculated after normalization to input and IgG controls. All antibodies used have previously been verified in ChIP. Quantitative RT–PCR Total RNA was extracted from cells at 75% confluence using the RNeasy mini kit (Qiagen). cDNA was then synthesized using SuperScriptIII reverse transcriptase (Life Technologies). qRT–PCR was performed using SYBR Green Master mix (Roche) and the ABI Prism 7300 Real Time PCR System (Applied Biosciences). Primer efficiency was verified by linear regression to a standard curve using 2, 1, 1/2, 1/4, 1/8, 1/16, 1/32, 1/64 and 1/128 dilutions. Reactions were carried out in quadruplicate at 95 °C for 10 min, followed by 40 cycles of 45 s at 95 °C and 45 s at 60 °C and 45 s at 72 °C. Values were standardized to housekeeping gene expression (ACTIN and HPRT); data were analysed using the comparative C t method. Murine L1 was amplified using primers (forward: 5′-ATGGCGAAAGGCAAACGTAAG-3′; reverse: 5′-ATTTTCGGTTGTGTTGGGGTG-3′). L1 in human cells was amplified using primers (5′-TGGAGGCATCACACTACCTG-3′; reverse: 5′-ATGCFFCATTATTTCTGAGG-3′). Bisulphite analysis Genomic DNA was purified from WT and SIRT6 KO MEFs and then exposed to the bisulphite conversion reaction using the EZ DNA Methylation kit (Zymo Research), following the manufacturer’s protocol. Following bisulphite conversion, relative methylation was quantified using bisulphite specific primers. Primers: L1 bisulphite forward: 5′-TAGGAAATTAGTTTGAATAGGTGAGAGG-3′, L1 bisulphite reverse: 5′-CCAAAACAAAACCTTTCTCAAACACTATA-3′. As a negative control, we confirmed that these primers did not amplify untreated genomic DNA. These primers have been previously described [51] . Micrococcal nuclease assay Micrococcal nuclease treatments were performed using the EZ Nucleosomal DNA Prep Kit (Zymo Research) as per the manufacturer’s protocol. In brief, mammalian nuclei were isolated from tissue culture cells and treated with 0.1, 0.25 and 0.5 U (unit) micrococcal nuclease for the 20 min at 42 °C. DNA was subsequently resolved in a 2% agarose gel. All experiments were performed in triplicate and a representative experiment is shown. In vitro assays In vitro mono-ADP ribosylation experiments were conducted essentially as previously described [19] . In brief, 5 μg of bacterially purified SIRT6 was incubated with 5 μg of the bacterially purified target substrate for 6 h in the presence of 32 P-NAD + . Transfer of the radiolabel by SIRT6 to the target substrate was used to quantify mono-ADP ribosylation activity. For the in vitro IP reaction, 5 μg of KAP1 was incubated with or without 5 μg of SIRT6 for 6 h before the addition of PCR-amplified L1 5′-UTR and 5 μg of HP1α. After 1.5 h, KAP1 was immunoprecipitated from the in vitro reaction and its affinity for HP1α was quantified using immunoblot. L1 5′-UTR sequence was generated by PCR using primers (forward: 5′-AATAGGAACAGCTCCGGTCTACAGCT-3′; reverse: 5′-AGCCTAACTGGGAGGCACCC-3′). ChIP-seq analysis We used the Human SIRT6 ChIP-seq data set (EMBL accession code SRX186647) to measure the magnitude of SIRT6 binding to L1 by comparing the frequency of reads derived from L1 repeats to all other sequences recovered via ChIP-seq. We first filtered the 36 bp ChIP-seq reads to exclude those that had any ambiguous characters. We then determined the set of unique reads (36mers) present in this data set and calculated the frequency of each. The vast majority of sequences appeared exactly once. We excluded these reads from subsequent analysis of read frequency to exclude any unique reads generated by sequencing error, creating a final set of 2,548,326 unique sequences. This also has the effect of making our measure of frequency more conservative. We then decomposed the sequences amplified by our L1 5′-UTR and 5′ CpG primers into all possible 36mers and calculated the frequency of each in the filtered set of reads. To examine the distribution of read depth across L1 elements, we performed a reference alignment of SIRT6 ChIP-seq reads to a full-length L1 sequence (Genebank accession code AF148856 ) using burrows-wheeler aligner (BWA) [52] . We used a quality filter of 20 and allowed for two mismatches. As the vast majority of L1s in the human genome are 5′ truncated (average L1 length is ~900 bp, 90–95% of all L1s are 5′ truncated), this analysis was unsurprisingly skewed towards the 3′ end of L1s. To correct for this bias, and to gain insight into SIRT6 depth across full-length L1s, we normalized the raw read depth by dividing the raw read depth for each nucleotide position by the relative abundance of truncated L1s that contain the given nucleotide position. In that way, our normalized depth provides insight into SIRT6 occupancy across only full-length L1s. Multiple reports have described the ratio of human L1s that are truncated, we used these reports as the basis for adjusting raw read depth to normalized read depth [53] , [54] . To understand the extent to which KAP1 and SIRT6 co-occupied promoters, we downloaded and compared all well-annotated target genes for each sequence from publically available data sets [54] , [55] . Single-cell genomic qPCR MEFs were generated from SIRT6 KO and WT embryos. These cells were subject to an equal number of passages during cell line expansion before analysis for new L1 insertions. Cell cycle arrested MEFs were then plated, one cell per well, in 96-well qPCR trays. By using cell cycle synchronized cells, derived from littermate embryos, that had been subject to the same number of passages, we reduced potential artefacts generated by DNA replication and differing amounts of cell divisions. qPCR was performed essentially as described previously [27] . In brief, primers targeting ORF2 (forward: 5′-ctggcgaggatgtggagaa-3′; reverse: 5′-cctgcaatcccaccaacaat-3) were used to amplify a 55-bp product. Control primers targeted non-mobile 5S ribosomal RNA sequence (forward: 5′-acggccataccaccctgaa-3′ and reverse: 5′-ggtctcccatccaagtactaacca-3′). Relative genomic ORF2 content was normalized to 5S genomic content. Sixty wells were used for each sample, the experiment was performed three times, with different mice contributing cells for each repeat. Co-immunoprecipitation HDF or MEF cells were harvested and lysed in IP lysis buffer (20 mM HEPES, pH 8.0, 0.2 mM EDTA, 5% glycerol, 150 mM NaCl and 1% NP40). The lysates were sonicated at 50% duty for 30 s followed by centrifugation for 10 min at 13,000 r.p.m. at 4 °C. The supernatants were then precleared by incubating them with 50% protein A agarose (Pierce, cat. no. 20333) for 1 h at 4 °C. The indicated primary antibody was added to the supernatants for overnight incubation at 4 °C, followed by incubation with protein A sepharose for 2 h. The beads were then spun down for 1 min at 8,000 r.p.m. at 4 °C and washed five times with IP lysis buffer. The proteins were eluted with 2 × sample buffer (Laemmli buffer:beta-mecaptoethanol=950:50) by boiling for 10 min, spun down and the supernatants were collected and used for western blotting with the indicated antibody. Input was loaded at 5%. Where indicated, samples were treated with 50 μg ml −1 ethidium bromide on ice for 30 min. Uncropped images of important immunoblots are shown in Supplementary Fig. 19 . Statistical tests Unless indicated otherwise, the Student’s t -test was used to determine whether differences between groups were statistically different. We set P values <0.05 as a threshold for statistical significance. How to cite this article : Van Meter, M. et al. SIRT6 represses LINE1 retrotransposons by ribosylating KAP1 but this repression fails with stress and age. Nat. Commun. 5:5011 doi: 10.1038/ncomms6011 (2014).